Control of exciton spin statistics through spin polarization in organic optoelectronic devices Spintronics based on organic semiconductor materials is attractive because of its rich fundamental physics and potential for device applications. Manipulating spins is obviously important for spintronics, and is usually achieved by using magnetic electrodes. Here we show a new approach where spin populations can be controlled primarily by energetics rather than kinetics. We find that exciton spin statistics can be substantially controlled by spin-polarizing carriers after injection using high magnetic fields and low temperatures, where the Zeeman energy is comparable with the thermal energy. By using this method, we demonstrate that singlet exciton formation can be suppressed by up to 53% in organic light-emitting diodes, and the dark conductance of organic photovoltaic devices can be increased by up to 45% due to enhanced formation of triplet charge-transfer states, leading to less recombination to the ground state. In the past few decades, optoelectronic devices based on organic semiconductors have been intensively investigated, and great success has been achieved in organic light-emitting diodes (OLEDs) [1] and organic photovoltaics (OPVs) [2] . In these devices, formation of neutral states through charge recombination has a crucial role in determining device efficiency [1] , [3] ; however, it is difficult to control this process directly. In OLEDs, simple models based on spin statistics predict that recombination of injected electrons and holes forms singlet and triplet excitons with a ratio of 1:3. Owing to weak spin–orbit coupling in most organic semiconductors, only singlet excitons contribute to light emission. By injecting spin-polarized carriers from magnetic electrodes, it is in principle possible to control the exciton spin statistics and light emission in OLEDs; however, only weak effects have been observed in this type of device [4] , [5] , [6] , [7] . The reason remains unclear, but is likely because of the difficulty of obtaining selective spin-polarized injection at metal/organic semiconductor interfaces [5] , [8] . When electrons are injected into an organic semiconductor device from the electrodes, they form a dilute non-degenerate system and thermal statistics should apply once the spin population has had time to equilibrate (in the absence of spin-selective recombination processes). Therefore, spin polarization can be an important effect in organic semiconductors devices at very low temperatures and high magnetic fields. In this case, the spins of electrons and holes will be aligned with the external magnetic field. For perfect spin alignment, only the ↓↓ triplet state can be formed when an electron and hole recombine, hence in high magnetic fields singlet state formation should be suppressed and triplet excitons preferentially formed; however, this effect has not previously been reported. Here we show a new approach that allows large changes in exciton spin statistics to be achieved by spin-polarizing carriers after injection using high magnetic fields and low temperatures, where the Zeeman energy is comparable with the thermal energy. By using this method, we demonstrate that the singlet formation can be suppressed by up to 53% in OLEDs, and the dark conductance of OPV devices can be increased by up to 45% due to enhanced formation of triplet charge-transfer (CT) states, leading to less recombination to the ground state. In addition to providing a sensitive test of the effects of spin-dependent recombination in OLEDs and OPVs, our high-field measurements confirm the importance of spin-dependent recombination in driving the smaller room-temperature magnetic field effects previously seen in these devices at low fields. Although the microscopic physics of spin polarization is simple, it is surprising that spin polarization translates into such large changes in macroscopic observables such as current and light output. These effects have not been observed in inorganic semiconductor spintronic devices, and rely on the unique physics of organic semiconductors. Light-emitting diodes To investigate the effects of spin polarization on recombination ( Fig. 1 ), we first performed experiments on typical OLED devices. We focus on high-efficiency polymer LEDs based on poly(9,9-dioctylfluorene-co- N -(4-butylphenyl)diphenylamine) (TFB) blended with poly(9,9-dioctylfluorene-co-benzothiadiazole) (F8BT). [9] The device structure was indium-tin oxide (ITO)/poly(3,4-ethylenedioxythiophene):poly(styrenesulfonate) (PEDOT:PSS, 40 nm)/TFB:F8BT (250 nm)/Ca (15 nm)/Al (100 nm). The TFB:F8BT layer was spin-coated from a 1:1 weight ratio solution in xylene (mixed isomers, 28 mg ml −1 ), followed by thermal evaporation of Ca and Al. We note the thick polymer layer used here is to maximize the spin-polarization effect by giving the carriers more time before recombination occurs. Device performance is shown in Supplementary Figs S1 and S2 . 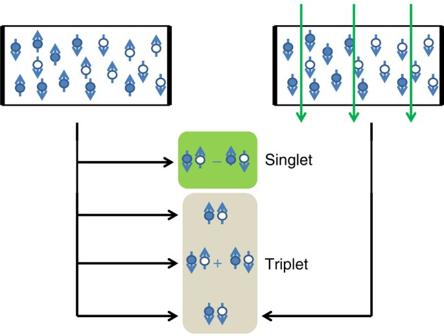Figure 1: The spin polarization effect in an organic optoelectronic device. Without applying an external magnetic field, electrons and holes have random spin orientations, and singlet and triplet excitons are formed in a ratio of 1:3. By applying a magnetic field at low temperature, the spins of electrons and holes will be aligned with the external magnetic field. The magnetic field direction is denoted by green arrows. For perfect spin alignment, only the ↓↓ triplet state can be formed when an electron and hole recombine. Figure 1: The spin polarization effect in an organic optoelectronic device. Without applying an external magnetic field, electrons and holes have random spin orientations, and singlet and triplet excitons are formed in a ratio of 1:3. By applying a magnetic field at low temperature, the spins of electrons and holes will be aligned with the external magnetic field. The magnetic field direction is denoted by green arrows. For perfect spin alignment, only the ↓↓ triplet state can be formed when an electron and hole recombine. 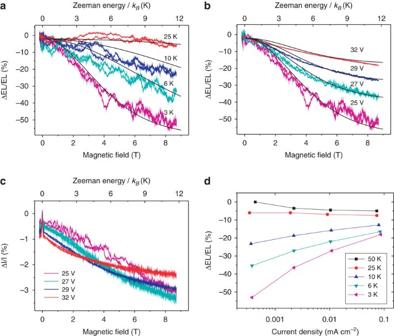Figure 2: Magnetic field effects in a TFB:F8BT LED. (a) Fractional change in EL as a function of magnetic field under constant biases at various temperatures, as indicated in the figure. The bias voltages are chosen to give a current density of ~4 × 10−4mA cm−2at zero magnetic field. The black curves are fits to the model described in the text. (b) Fractional change in EL as a function of magnetic field at 3 K under various bias voltages. The black curves are fits to the model described in the text. (c) MC at 3 K under various bias voltages. (d) Fractional change in EL as a function of current density at 8.7 T at various temperatures. Here the current density is the zero-field value, and the device is under constant bias voltage during the measurement. Full size image Figure 2a shows the change of device electroluminescence (EL) at constant biases as a function of magnetic field at various temperatures. Here different constant bias voltages are chosen at different temperatures to ensure similar zero magnetic field current densities (~4 × 10 −4 mA cm −2 ). It shows that the EL intensity decreases when the applied magnetic field increases, and this effect increases dramatically when the temperature decreases. The amount of EL quenching becomes as high as 53% at 3 K and 8.7 T. Figure 2b shows the change of EL at various constant biases as a function of magnetic field at 3 K. At high bias, the EL quenching effect is significantly reduced. During the measurement, the device current only changes slightly (~3%), as shown in Fig. 2c . Figure 2d summarizes the EL quenching effect under various driving conditions at 8.7 T and at different temperatures; detailed data are given in Supplementary Fig. S3 . Figure 2: Magnetic field effects in a TFB:F8BT LED. ( a ) Fractional change in EL as a function of magnetic field under constant biases at various temperatures, as indicated in the figure. The bias voltages are chosen to give a current density of ~4 × 10 −4 mA cm −2 at zero magnetic field. The black curves are fits to the model described in the text. ( b ) Fractional change in EL as a function of magnetic field at 3 K under various bias voltages. The black curves are fits to the model described in the text. ( c ) MC at 3 K under various bias voltages. ( d ) Fractional change in EL as a function of current density at 8.7 T at various temperatures. Here the current density is the zero-field value, and the device is under constant bias voltage during the measurement. Full size image Generally, changes in EL intensity with magnetic field (MEL) can be caused by changes in the following factors: (i) carrier mobility [10] , (ii) recombination rates [11] , (iii) formation ratio of singlet and triplet states, (iv) intersystem crossing (ISC) [12] and (v) triplet–triplet annihilation (TTA) [13] , [14] . As the device current changed only slightly ( Fig. 2c ), changes in carrier mobility are insufficient to explain the large observed MEL. Direct enhancement of recombination rates via singlet and triplet pathways has been proposed to explain the positive MEL effects seen by Reufer et al. [15] , but cannot explain the large negative MEL seen here. Spin mixing in organic semiconductors can be caused by the hyperfine coupling (HFC) [16] , [17] and Δg mechanisms [18] , [19] . Before forming intramolecular excitons, intermolecular CT states are formed through electron-hole recombination. ISC can occur much more easily in CT states than in tightly bound intramolecular excitons, because the CT states have much smaller exchange energy. By applying an external magnetic field which is comparable to the hyperfine field, HFC can be suppressed and ISC is reduced, thus reducing the overall recombination rate from CT states. These effects have been extensively investigated in OLEDs (see for example Hu et al. [12] , Dediu et al. [20] and Kersten et al. [21] ). In our measurement, we also observe a small reduction in EL (~1%) at magnetic fields up to 0.1 T. However, changes in ISC caused by HFC will saturate at relatively small magnetic fields, and therefore cannot explain our large-field results. Also, ISC caused by the Δ g mechanism is expected to increase ISC at high field [19] , and then it will produce a positive MEL, in contrast to the negative MEL that we observe. Therefore, magnetic field dependence of ISC is not the reason for the observed large negative MEL at high magnetic fields. It has been shown that additional singlet excitons can be produced through TTA, and TTA can be suppressed by high magnetic fields, which results in a negative MEL [13] , [14] . In fact, the TTA process becomes important only when the excitation density is high [13] , [14] . In our measurement, we observe that the MEL is more significant at lower carrier density when the temperature is below 10 K. Therefore, we believe that TTA does not play a significant role in the lowest current density case. At 50 K, the MEL slightly increases at higher current densities ( Fig. 2d ), which indicates that TTA might play a role under these conditions. In addition, the maximum MEL expected due to modulation of TTA is 37.5% (ref. 22 ), smaller than the effect that we observe. On the basis of the above analysis, we believe that the observed large MEL at low bias is caused directly by the magnetic field dependence of the formation probabilities of singlet and triplet states. At high magnetic field and low temperature, the Zeeman energy is comparable to the thermal energy (for example, the Zeeman energy is about 60 μeV at 1 T, and the thermal energy is about 250 μeV at 3 K), and then the spin polarization effect becomes important if the charge carriers have had time to relax before recombination. In this case, fewer singlet states and more triplet states will be formed, which directly results in EL quenching. To set up a simple model for this process, we assume that the equilibrium spin populations are determined by Boltzmann statistics corresponding to the Zeeman energy, and that the populations relax exponentially to this equilibrium state with a characteristic time τ s . We assume that the carriers are unpolarized on injection, and that they recombine in a well-defined carrier recombination time τ c that is the same for electrons and holes. Pairs of parallel spins are assumed to recombine to triplet states, and antiparallel spins recombine to singlet or triplet states with equal probability. The detailed calculation is shown in Supplementary Methods . Applying the model to the 3 K data in Fig. 2a gives a good fit with a ratio τ c / τ s of 1.43. In the absence of independent measurements of τ c / τ s , we fit the temperature-dependent data in Fig. 2a with the same value of τ c / τ s ; a reasonable fit to the magnitude and shape of the MEL effect as a function of temperature is obtained. Figure 2b displays fits of the MEL at various bias voltages at 3 K, here allowing τ c / τ s to vary. Values of τ c / τ s of 1.43, 0.95, 0.72 and 0.50 are obtained at voltages of 25, 27, 29 and 32 V, respectively. The clear decrease in τ c / τ s as the bias voltage increases is consistent with a reduced charge–carrier lifetime due to the larger electric field and higher mobility (due to its dependence on field and carrier density), possibly assisted by a higher bimolecular recombination rate at higher bias (or high current density). The τ c / τ s value can also be tuned by changing device thickness, and we indeed observe that thinner devices have smaller MEL ( Supplementary Fig. S4 ). The observed deviations of the MEL data from the model at high biases are likely due to the TTA process playing a role when the current density is high. To obtain independent validation of our model, we can estimate τ s by measuring the transient EL after turning on the device (see Supplementary Fig. S5 ). The initial EL is insensitive to magnetic field, and the MEL effect builds up on a characteristic timescale of ~150 μs, independent of temperature. The additional carriers that are injected are initially almost unpolarized, and the time taken for the magnetic field effect to build up is thus a direct measure of τ s . The value of τ c is more difficult to measure independently, due to the dispersive nature of transport and recombination, and the presence of two carrier types in the device. We note that the EL overshoot after turn-on stabilizes on a timescale of about 75 μs, and this provides one measure of a characteristic timescale for transport and recombination that agrees with the τ c / τ s ratio determined by fitting the MEL data above. Smaller or larger values of τ c can, however, be estimated respectively from the fast EL turn-on or from mobilities extracted assuming space–charge-limited currents. Broadly, our independent measurements of τ c and τ s conclude that they are of the same order, consistent with the τ c / τ s ratios that we extract from fitting the MEL data. We note that in F8BT:TFB devices the singlet CT states initially formed by electron-hole recombination relax to form bound emissive CT states (sometimes termed exciplexes) at the F8BT/TFB interface [9] . At low temperatures, the EL comes predominantly from these singlet exciplex states [9] . This contrasts with LEDs based on a single polymer, where intermolecular singlet CT states relax to form intrachain singlet excitons. In both cases triplet CT states relax rapidly to the lower-energy intrachain triplet exciton, which is non-emissive. In the absence of significant dissociation or spin mixing of the emissive state the MEL effect should be independent of whether the emission is from an intrachain or inter-chain singlet state. This is confirmed by the fact that we also observe MEL effects (of similar magnitude to those described above) in single-polymer LEDs based on poly(9,9-dioctylfluorene) (F8) and poly(2-methoxy-5-(2′-ethyl-hexyloxy)- p -phenylene vinylene) (see Supplementary Fig. S6 ). Photovoltaic devices We have shown that the spin statistics can be controlled in OLED devices at high magnetic fields, with very obvious effects on optical emission. In general, changing the spin statistics can change the net rate of recombination, and this can change the current flowing in the device, leading to magnetoconductance (MC) effects [19] , [23] , [24] , [25] . However, in the devices studied above these effects are small, probably because the tightly bound exciplex or exciton states formed by recombination are unlikely to be redissociated to form free charges. Instead, they will rapidly relax to the lower-energy intrachain triplet exciton state, as shown in Fig. 3a . Hence, although the population of charge pairs will increase as the recombination rate is reduced, this will not have a direct effect on the population of free charges responsible for the current. In other systems, however, particularly those that operate efficiently as photovoltaics, dissociation of charge pairs is an important process in competition with recombination, and significant effects on the electrical properties might be expected by changing the net recombination rate [25] , [26] . We therefore now examine MC effects in the dark current of OPV devices. One good example is a typical poly(3-hexylthiophene):[6,6]-phenyl-C 61 -butyric acid methyl ester (P3HT:PCBM) OPV system. In this system, the intrachain triplet exciton is a higher-energy state [27] than the CT state, therefore the long-lived triplet CT states can be dissociated to become free changes and contribute to device current, and a significant MC effect is expected when charge carriers are spin polarized, as shown in Fig. 3b . 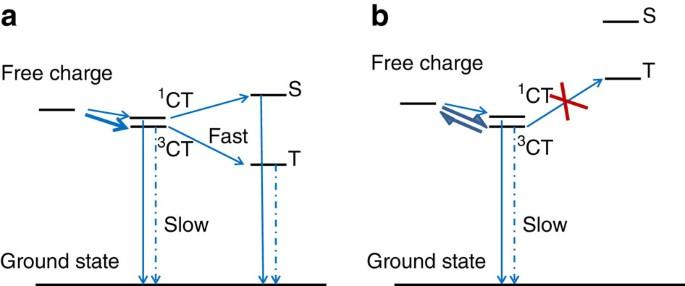Figure 3: Schematic of recombination pathways and timescales. Spin polarization due to the magnetic field changes the ratio of singlet and triplet charge-transfer states (1CT and3CT, respectively) formed by charge recombination, as shown inFig. 1. For the LED device (a), triplet CT states recombine rapidly to form lower-energy triplet excitons. For the photovoltaic device (b), the triplet exciton state is higher in energy than the triplet CT state. Triplet CT states therefore have a long lifetime and can be redissociated to form free charges. This leads to a net free-charge recombination rate that depends on the magnetic field. T and S denote triplet and singlet excitons, respectively. Figure 3: Schematic of recombination pathways and timescales. Spin polarization due to the magnetic field changes the ratio of singlet and triplet charge-transfer states ( 1 CT and 3 CT, respectively) formed by charge recombination, as shown in Fig. 1 . For the LED device ( a ), triplet CT states recombine rapidly to form lower-energy triplet excitons. For the photovoltaic device ( b ), the triplet exciton state is higher in energy than the triplet CT state. Triplet CT states therefore have a long lifetime and can be redissociated to form free charges. This leads to a net free-charge recombination rate that depends on the magnetic field. T and S denote triplet and singlet excitons, respectively. Full size image The OPV device structure was ITO/PEDOT:PSS (40 nm)/P3HT:PCBM (100 nm)/Al, and the P3HT:PCBM layer was spin-coated from a 5:4 weight ratio solution in chlorobenzene (20 mg ml −1 ). Device characteristics are shown in Supplementary Figs S7 and S8 . 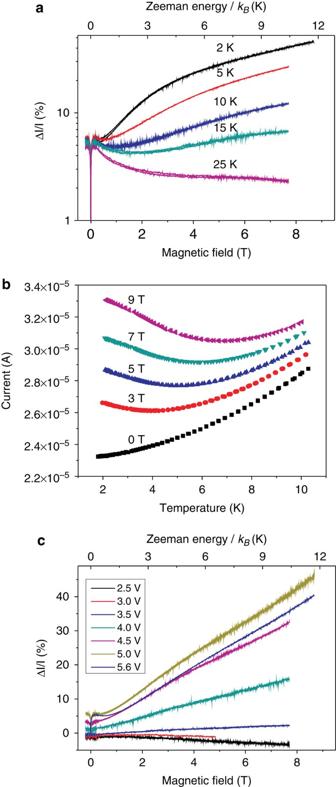Figure 4: MC in an P3HT:PCBM device. (a) MC (on a logarithmic scale) under constant bias at various temperatures. The zero magnetic field current density is always ~0.5 mA cm−2. (b) Device current as a function of temperature under constant 5.0 V bias at various magnetic fields. (c) MC at 2 K under various bias voltages. Figure 4a shows the MC on a logarithmic scale as a function of magnetic field at various temperatures. These measurements were performed with similar zero-field current densities of ~0.5 mA cm −2 . As seen above, the MC rises rapidly at low magnetic fields (<0.1 T), but then appears to saturate. This small-field effect is similar to that seen in the literature [16] , [19] , [25] , [28] , which is due to changes in HFC-induced ISC. However, when the magnetic field increases further, a new and significant MC effect appears at low temperatures. At 2 K, we observe a positive MC as high as 45% at 8.7 T. This positive high-field MC effect decreases rapidly with increasing temperature, becoming negative at 25 K. Figure 4b shows the temperature dependence of the device current under constant bias voltage at various magnetic fields. Detailed data at different temperatures are given in Supplementary Figs S9 and S10 . At zero magnetic field, the device current decreases monotonically with decreasing temperature. At 3 T, the current begins to increase as the temperature falls below 4 K. The point of minimum conductivity moves to higher temperatures as the magnetic field increases, reaching a temperature of approximately 6.5 K at 9 T. These results are surprising, as the temperature dependence appears to switch from that expected for hopping conduction to that expected for metallic conduction as the magnetic field is increased. The fact that the MC behaviour is so similar to the MEL in OLED devices leads us to consider that the MC may also be caused by the spin-polarization effect. Figure 4: MC in an P3HT:PCBM device. ( a ) MC (on a logarithmic scale) under constant bias at various temperatures. The zero magnetic field current density is always ~0.5 mA cm −2 . ( b ) Device current as a function of temperature under constant 5.0 V bias at various magnetic fields. ( c ) MC at 2 K under various bias voltages. Full size image There are a number of other commonly considered high-field MC mechanisms for devices based on non-magnetic materials. These include: classical MC caused by the Lorentz force; hopping MC due to wavefunction shrinkage [29] ; weak localization due to quantum interference [30] ; and bipolaron formation [10] , [31] . The first two mechanisms can be ruled out in our devices because they result only in negative MC effects. MC caused by the weak localization effect and bipolaron formation might be positive. However, all these mechanisms are single-carrier effects that should be present in electron-only or hole-only devices. As shown in Supplementary Fig. S11 , the MC effects in these single-carrier devices are very much suppressed, and become almost unobservable. Therefore, we can also rule out weak localization and bipolaron formation effects in our system. Hence, we return to changes in the recombination process due to spin polarization as the dominant mechanism to explain the observed large MC effect. In OPVs, CT states can be formed through bimolecular recombination following injection of electrons and holes from electrodes. Singlet CT states will recombine quickly to the ground state, whereas triplet CT states will recombine more slowly. Relaxation of triplet CT states to form intramolecular triplet excitons can in some cases provide an additional pathway for removal of triplet CT states, but in this system the CT state is sufficiently low in energy that this process is forbidden [27] . Thus, triplet CT states are more likely than singlets to be redissociated into free charges, and enhanced formation of triplet CT states will therefore reduce the net recombination rate for free charges. In our measurements, it is the enhanced formation of triplet states due to spin polarization that we believe is responsible for the large observed MC. As discussed by Bergeson et al. [24] in the low-field regime where changes in recombination rate are also observed, the effect of these changes on the measured current is complex, and the sign and intensity of the MC are sensitive to the exact driving conditions. In our devices, as shown in Fig. 4c , at 2 K we observe a positive MC at biases above 3.5 V where the injected current is significant. In this regime, recombination must be in competition with electrons and holes passing through the device without recombination, such that reducing the recombination rate increases the measured current. At higher bias, the MC tends to saturate and starts to decrease at biases above 5 V ( Fig. 4c ). This may be due to changes in the competition between carrier recombination and extraction at high biases, or due to the reduced time available for spin polarization to occur before recombination at higher bias. The role of spin-dependent recombination in organic devices is still controversial, and our technique allows models for device operation to be tested by achieving direct control of spin populations in a manner that is controlled primarily by energetics rather than kinetics. Our results are consistent with spin-dependent recombination being the dominant effect explaining low-field magnetic field effects in organic devices, although the amount by which recombination influences the current can vary greatly from system to system depending on the relative energies of CT states, singlet excitons and triplet excitons. In the high-field regime where spin polarization occurs, we see strong changes in the EL with magnetic field, even when the changes in the current are small. The strong spin polarization effects that we observe are unique to organic semiconductors, as they are free from the Pauli paramagnetism effects, high doping densities and strong spin–orbit coupling typically present in inorganic semiconductor devices. By spin-polarizing carriers in polymer-based devices, we have shown that the EL can be suppressed by as much as 53% in OLEDs, and the dark current can be increased by 45% in OPVs. Device preparation After being cleaned and oxygen plasma-treated, ITO-coated glass substrates were spin-coated with a layer of 40 nm-thick PEDOT:PSS, and then were annealed at 150 °C for 10 min under nitrogen gas flow before being transferred to a nitrogen glove box for further fabrication processes. For LED devices, the TFB:F8BT layer was spin-coated from a 1:1 weight ratio solution in xylene (28 mg ml −1 , mixed isomers), and the active layer formed is ≈250 nm thick. Microscopic phase separation is observable on lengthscales of about 2–5 μm, but there is significant intermixing of the two components within these phases. Calcium and aluminium were deposited on top of the polymer layer by thermal evaporation through a mask, which defined an active area of 4.5 mm 2 . The device showed an LED efficiency at room temperature of 3.1 cd A −1 at a luminance of 100 cd m −2 . For PV devices, the P3HT:PCBM layer was spin-coated from a 5:4 weight ratio solution in dichlorobenzene (20 mg ml −1 ), and the active layer formed is approximately 100 nm thick. Aluminium was deposited on top of the P3HT:PCBM layer by thermal evaporation through a mask, which defined an active area of 4.5 mm 2 . After the deposition, thermal annealing was performed at 140 °C for 5 min in the glove box. The devices showed a good solar cell power conversion efficiency at room temperature of 3.9% (see Supplementary Fig. S7 ). The devices were briefly (~5 min) exposed to the air when they were transferred to a cryostat for MC measurement. To fabricate single-carrier devices, all the procedures were the same as those for the normal devices, except that different top and bottom contacts were chosen so that electrons or holes could be blocked effectively. For the hole-only devices, the aluminium top electrode in the normal device structure was replaced by evaporated palladium (50 nm) [32] . Palladium successfully suppresses the electron injection into PCBM due to the large energy barrier. For electron-only devices, the ITO/PEDOT:PSS bottom contact was replaced by silver (Ag, 50 nm)/self-assembled monolayer (SAM) [32] . 1-decanethiol (CH 3 (CH 2 ) 9 SH, purity 99% from Sigma-Aldrich) was used as a suitable SAM layer for modifying the workfunction of the Ag electrode. A layer of 50 nm silver was evaporated on a glass substrate. After being kept in 1-decanethiol solution in 2-propanol (~3 mM) overnight, the substrates were thoroughly rinsed with 2-propanol to remove unbound SAMs and dried using nitrogen before spin coating of the active layer. Magnetic field effect measurement Magnetic field effect measurement was performed in a superconducting magnet with optical windows. A Keithley source-measure unit was used to supply the bias voltage and measure the current. Al was ground and ITO was anode. The EL emission was from the ITO/glass side. By using an external light source, the transmittance of ITO glass substrate transmittance was found to be independent of magnetic field from 2 K to room temperature. A set of lenses was used to enable the light emission from the device to be concentrated at a point, which was about 1.5 m away from the magnet. The sensitivity of Si-photodetector at this distance was not affected by the magnet; this was checked using an external light source. The magnetic field was perpendicular to the device substrate. The sweep rate for the magnetic field was 1 mT s −1 for B <0.2 T, 5 mT s −1 for 0.2 T< B <5 T and 3 mT s −1 for B >5 T. The device current was record during sweeping of the magnetic field. The device EL was detected using a high sensitivity Si photodiode. How to cite this article: Wang, J. et al. Control of exciton spin statistics through spin polarization in organic optoelectronic devices. Nat. Commun. 3:1191 doi: 10.1038/ncomms2194 (2012).